Inconsistent prediction capability of ImmuneCells.Sig across different RNA-seq datasets 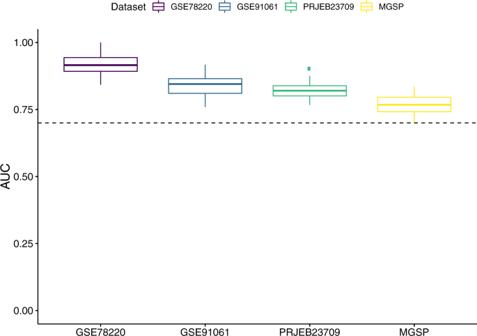Fig. 1: The predictive ability of a random gene set by using the same implementation scheme with Xiong et al.1on four melanoma datasets. Fifty random sampling of around 100 genes among total genes in each dataset were tested faithfully using the implementation provided by the original paper. The actual number of genes used is 103 for GSE78220 and GSE91061, 101 for PRJEB23709, and 98 for MGSP. Box plots show the median (center line), upper quartiles and lower quartiles with whiskers extend to 1.5x interquartile range. The dotted line is drawn at AUC value equal to 0.7. 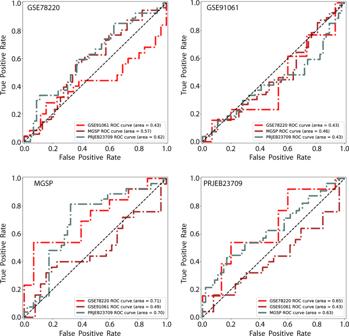Fig. 2: The performance of the ImmuneCells.Sig signature on predicting ICT outcomes in four melanoma patient datasets. For each ROC curve plot, the plot title refers to the training dataset for the predictive model, while the trained model was tested on the three remaining datasets. RNA-seq expression datasets We downloaded the preprocessed datasets GSE78220 [2] , GSE91061 [3] , PRJEB23709 [4] , and MGSP [5] directly from Xiong et al. [1] ( https://github.com/donghaixiong/Immune_cells_analysis ). The preprocess procedure in the original paper included three steps. First, the raw RNA-seq reads were aligned to the hg19 human reference genome using Bowtie-TopHat (version 2.0.4) [7] . Then, the gene expression read counts were obtained with the htseq-count Python script from HTSeq v0.11.1 ( https://htseq.readthedocs.io/en/release_0.11.1/ ). The read counts data were further transformed by regularized log (DESeq2 v1.28.1 [8] ). Testing with random gene sets shows the effect of overfitting The ImmuneCells.Sig signature was discovered from the scRNA-seq datasets [9] and a bulk gene expression dataset GSE78220 [2] . A nearest-centroid classifier [10] , [11] was then trained by cancerclass v1.32.0 R package [10] to predict ICT response using the identified signature. The performance of the prediction was then evaluated by the receiver operating characteristic curves (ROC) and the area under the ROC curve (AUC). To illustrate the effect of overfitting due to training and testing on the same dataset, we evaluated random gene sets with the same implementation. We randomly drew a set of genes from all the genes present in each gene expression dataset without considering their biological functions as a signature, and trained nearest-centroid classifiers individually on each dataset using the model fitting code provided by the original paper [1] . For fair comparison, the number of genes selected equals the number of genes of the ImmuneCells.Sig signature for each dataset, respectively (103 genes for GSE78220 and GSE91061, 101 genes for PRJEB23709, and 98 genes for MGSP). After 50 bootstrapping in all datasets, the highest AUC value could reach 1 for GSE78220, 0.917 for GSE91061, 0.902 for PRJEB23709, and 0.835 for MGSP (Fig. 1 ). The generalization capability of ImmuneCells.Sig To test the generalization capability of the ImmuneCells.Sig signature, we changed the prediction process such that one dataset was used for training a model with the original model fitting code without modification, while the remaining independent datasets were used for testing. The predictive models using ImmuneCell.Sig did not show robust prediction results (Fig. 2 ). In some cases, the testing AUC values were below 0.5.